Strongly correlated two-dimensional plasma explored from entropy measurements Charged plasma and Fermi liquid are two distinct states of electronic matter intrinsic to dilute two-dimensional electron systems at elevated and low temperatures, respectively. Probing their thermodynamics represents challenge because of lack of an adequate technique. Here, we report a thermodynamic method to measure the entropy per electron in gated structures. Our technique appears to be three orders of magnitude superior in sensitivity to a.c. calorimetry, allowing entropy measurements with only 10 8 electrons. This enables us to investigate the correlated plasma regime, previously inaccessible experimentally in two-dimensional electron systems in semiconductors. In experiments with clean two-dimensional electron system in silicon-based structures, we traced entropy evolution from the plasma to Fermi liquid regime by varying electron density. We reveal that the correlated plasma regime can be mapped onto the ordinary non-degenerate Fermi gas with an interaction-enhanced temperature-dependent effective mass. Our method opens up new horizons in studies of low-dimensional electron systems. Interaction between conduction electrons is well known to become more and more important as dimensionality is reduced and as carrier density decreases. Consequently, the dilute two-dimensional (2D) electron systems exhibit a variety of spectacular interaction effects such as the fractional quantum Hall effect [1] , metal–insulator transition (MIT) in 2D [2] , [3] , strong enhancement in the effective mass and spin susceptibility [4] , [5] and so on. The vast majority of these phenomena are explored using charge transport and Coulomb drag [6] measurements. The apparent simplicity of these techniques, however, is spoiled by an indirect character of the results whose interpretation requires specific theoretical models. In contrast, thermodynamic measurements carry more direct information on the electron–electron correlations. However, these measurements are harder because of the smallness of thermodynamic quantities for a dilute single-layer 2D system confining, typically, 10 8 –10 10 electrons. By now, only electron compressibility [7] , [8] , [9] , spin magnetization [10] and chemical potential [11] have been measured in low-density 2D carrier systems, whereas the major thermodynamic parameter—entropy—has never been explored. Here, we show how the entropy per electron, ∂ S /∂ n , can be measured for 2D electron systems ( n is the electron density). According to the Maxwell relation (∂ S /∂ n ) T =−(∂ μ /∂ T ) n , the sought for entropy is found from the temperature derivative of the chemical potential. To measure ∂ μ /∂ T of the 2D electron layer, we use a gated structure (shown schematically in Fig. 1a ) where the 2D electrons and the gate act as two plates of a capacitor. When temperature is modulated, the chemical potential of the 2D layer varies causing the capacitor recharging. 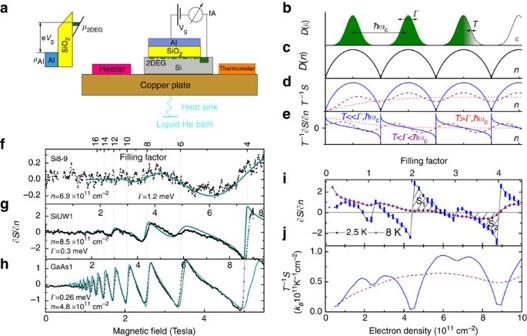Figure 1: Scheme of experiment and and entropy in perpendicular magnetic field. (a) Experimental set-up, schematic cross-section, and energy band diagram of the Si-MOSFET structure. (b,c) The density of states for a 2D electron gas in quantizing magnetic field versus energy and electron density, respectively. Green colour denotes filled states. (d,e) RatiosS/TandT−1∂S/∂nversus electron density for different relationships between Γ,Tandℏωc(shown in the figure). (f–h) The entropy per electron atT=3 K versus magnetic field measured with three samples ((f) Si8-9, (g) Si-UW1, and (h) GaAs1). The upper axis (filling factorν=eB/(hn) ) is common for all the three panels. The densities are shown on the panels. Cyan curves represent the fit using the noninteracting electron gas model with the band effective masses and level broadenings indicated on the panels. (i) ∂S/∂nversus density measured at 9 T with Si-UW2. The temperatures are shown on the panel. Hatched regions S1and S2have approximately the same area (see text). The data spread for each density at 2.5 K indicate typical noise level. (j) Normalized entropy versus density for the same sample. Figure 1: Scheme of experiment and and entropy in perpendicular magnetic field. ( a ) Experimental set-up, schematic cross-section, and energy band diagram of the Si-MOSFET structure. ( b , c ) The density of states for a 2D electron gas in quantizing magnetic field versus energy and electron density, respectively. Green colour denotes filled states. ( d , e ) Ratios S / T and T −1 ∂ S /∂ n versus electron density for different relationships between Γ, T and ℏ ω c (shown in the figure). ( f – h ) The entropy per electron at T =3 K versus magnetic field measured with three samples (( f ) Si8-9, ( g ) Si-UW1, and ( h ) GaAs1). The upper axis (filling factor ν = eB /( hn ) ) is common for all the three panels. The densities are shown on the panels. Cyan curves represent the fit using the noninteracting electron gas model with the band effective masses and level broadenings indicated on the panels. ( i ) ∂ S /∂ n versus density measured at 9 T with Si-UW2. The temperatures are shown on the panel. Hatched regions S 1 and S 2 have approximately the same area (see text). The data spread for each density at 2.5 K indicate typical noise level. ( j ) Normalized entropy versus density for the same sample. Full size image The experimental set-up is similar to the one used in ref. 10 for spin magnetization measurements. The sample (either Si-MOSFET or GaAs-FET) and the copper sample holder are kept in a thermal contact with a wire heater, which modulates their temperature: T ( t ) T 0 +Δ T cos( ωt ). In our experiments, temperature T 0 typically varies from 2.4 to 26 K, and is modulated at the frequency ω /(2 π )≈0.5 Hz with an amplitude Δ T ∼ 0.1–0.2 K. See Supplementary Note 1 for details concerning temperature modulation. Modulation of the sample temperature changes the chemical potential and, hence, causes recharging of the gated structure. Therefore, ∂ μ /∂ T is directly determined in the experiment from the measured recharging current: Here, C stands for the capacitance between the gate electrode and 2D electron layer. Both T 0 and Δ T values were measured using a miniature thermometer attached to the copper sample chamber and C was determined in the same experiment. Using the PPMS-9 cryomagnetic system, we applied magnetic field up to 9 T either parallel or perpendicular to the sample plane. We used the following four samples: a Schottky-gated GaAl/AlGaAs heterostructure (sample GaAs1) with peak mobility about 20 m 2 V −1 s −1 , and three Si-MOS structures (Si-UW1, Si-UW2 and Si8-9) with the peak mobilities ∼ 3 m 2 V −1 s −1 , 3 m 2 V −1 s −1 and 0.5 m 2 V −1 s −1 , respectively. For more details concerning the introduced measurement technique, see Supplementary Note 2 . Measurements in quantizing magnetic fields To test the technique, we start from measurements of ∂ S /∂ n in quantizing perpendicular magnetic fields. In strong fields, the energy spectrum of the system consists of a ladder of the broadened Landau levels whose density of states D ( ɛ ) is shown schematically in Fig. 1b . For simplicity, we focus on the cyclotron splitting ℏ ω c and neglect Zeeman splitting, and interaction effects. In the low-temperature limit (T<< ℏ ω c ,Γ, E F ) the entropy of the noninteracting 2D electron gas is given by where D = D ( ɛ = E F ) is the density of states at the Fermi energy. We use throughout the paper κ B =1. To find ∂ S /∂ n , we express D versus n (see Fig. 1c ) using the definition with f F ( ɛ )=1/[1+exp(( ɛ – μ )/ T )] being the Fermi–Dirac distribution function. The resulting anticipated behaviour of the entropy and ∂ S /∂ n as a function of n is plotted in Fig. 1d,e , respectively. We emphasize that the calculated entropy vanishes together with D in the gaps between Landau levels. As temperature increases and becomes larger than the level broadening Γ, the entropy dips get smeared (see Fig. 1d,e ) being averaged over energy interval ∼ T . Finally, in the high temperature limit T ≫ ℏ ω c , the level quantization is washed out and the entropy S ( n ) should approach the monotonic dependence anticipated for zero magnetic field (see below). In Fig. 1f–h , the calculated entropy is compared with the measured magnetic field dependence of ∂ S /∂ n for three different samples. The cyan curves show a fit (for details of the fit see Supplementary Note 3 ) of the data with the theoretical model (given in Supplementary Note 4 ) for noninteracting electrons using a bare band mass and a realistic level broadening. The data for the most disordered sample Si8-9 demonstrates only cyclotron gaps resolved at the filling factors ν =4 and ν =8 ( for (100) Si-MOS structures, the 2D electron layer has additional twofold valley degeneracy). To fit the data at ν =6 (spin gap) for the clean sample Si-UW1, we used an enhanced g-factor g eff =4. As known, enhancement of the spin gap due to the inter-level exchange interaction is a precursor of the quantum Hall ferromagnetism [12] . The good agreement of the data for GaAs1 sample with the noninteracting theory ( Fig. 1h ), allows us to compare our method with the state-of-the-art AC calorimetry performed with similar GaAs-samples [13] . It appears that our technique has three orders of magnitude higher resolution than the AC calorimetry (see Supplementary Note 5 ). Importantly, it is also free from the lattice specific heat contribution. We now consider the interacting 2D electron system in Si-MOSFET samples. Since the density of states in the middle of the gap (at ν =2 or ν =4) is negligibly small, the entropy at both points should be close to zero. This implies that the area S 1 (positive signal) and area S 2 (negative signal) should completely compensate each other, as shown in Fig. 1i . This integral property is not affected by correlation effects and is fulfilled in the experimental data with a good accuracy. We can now evaluate the entropy of the system: In the ideal case, for integration one would have to choose n 0 =0 where S (0)=0 by definition. However, the 2D system can never be fully depleted: below a threshold density n th it becomes nonconducting and fails to recharge. For our temperature range T >2.5 K and in magnetic fields B <1 T, we could deplete the samples Si-UW1 and Si-UW2 down to densities n th ∼ 3 × 10 10 cm −2 , which correspond to ∼ 1 GOhm resistance of the 2D electron system. Therefore, in a strong magnetic field, it is more practical to choose n 0 as the initial point for the integration such that it corresponds to an even filling factor ( ν =2 or 4 in our case) where the gap is large. This choice ensures the S ( n 0 ) value to be close to zero. The integrated entropy is shown in Fig. 1j . As expected from Fig. 1i , at even filling factors ( ν =0,2,4) the entropy is almost zero. This fact supports our method of entropy reconstruction. Measurements in zero perpendicular field We now turn to more delicate thermodynamic effects for the 2D electron system in zero perpendicular field. For noninteracting 2D electron gas with a simple parabolic spectrum ( ɛ = p 2 /2 m b ), the density of states is constant D = g s,v m b /2 π ℏ 2 . Here g s,v denotes the total (spin and valley) spectrum degeneracy, and m b is the band mass (for (100)Si-MOS g s,v =4, and m b ≈0.2 m e ; ref. 14 ). In the degenerate limit E F =n/D ≫ T , the entropy S = πT g s,v m b /6 ℏ 2 is independent of density, ∂ S /∂ n =0, with the exponential accuracy. In the opposite limit E F << T , the temperature is the dominant parameter and the entropy per electron agrees with that for the ideal Boltzman gas ∂ S /∂ n ∝ ln( n / T ). For arbitrary temperature, the well-known result for a noninteracting 2D electron gas is given as With high-mobility Si-MOSFET samples, in contrast to the ubiquitous charge transport, our thermodynamic technique provides an access to the very dilute regime n ∼ (3 × 10 10 –10 11 ) cm −2 . For such low densities and interaction-enhanced quasiparticles effective mass m * ∼ (0.4–0.6) m e one can readily enter the non-degenerate regime T > E F . Moreover, in this regime, the typical electron–electron interaction energy is about several meV, that is, an order of magnitude higher than both temperature and the Fermi energy ( κ ≈7.7 is the effective dielectric constant for the Si/SiO 2 interface) [14] . Such strong interaction modifies the spectrum and brings us to an unexplored [15] regime of a correlated 2D charged plasma. In the low-temperature Fermi-liquid (FL) regime, the zero field entropy is given by equation (2) in which D is replaced by the density of quasiparticle states at the Fermi level, D *=g s,v m */(2 π ℏ 2 ) (ref. 16 ). In contrast to the noninteracting case, D * depends on the electron density n via the effective mass m *( n ), which includes renormalization due to electron–electron interaction. Then one finds from equation (2) that ∂ S /∂ n =[ πTg s,v /(6 ℏ 2 )] ∂ m */∂ n ; this relates the measured quantity to the ∂ m */∂ n . In this regime, the density derivative of the entropy is expected to be negative (see insert to Fig. 2a ) since electron–electron interaction increases the effective mass, ∂ m */∂ n<0 (ref. 4 ). 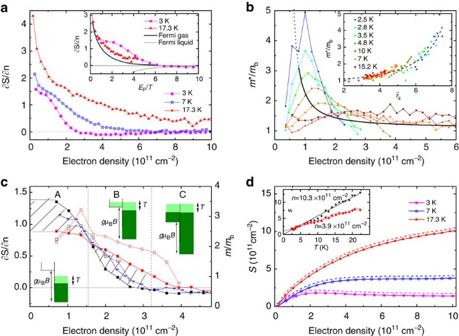Figure 2: Entropy per electron in zero perpendicular field. (a) The entropy per electron ∂S/∂nversus density (symbols) for various temperatures, sample Si-UW2. Inset: the same data versus dimensionless density (EF/T), the solid curve is the expectation for the Fermi gas with the Si band parameters, the dashed curve is the expectation for the FL with negative ∂m*/∂n(see text); (b) the effective massm* versus density. The black curve corresponds to the approximation ofm* from the Shubnikov-de-Haas measurements4. Symbols are them*(n,T) data determined using equation (4) from the measured ∂S/∂nvalues. Different symbols correspond to different temperatures (shown in the inset). Scaling of the effective mass versus effective interaction parameteris shown in the inset(see text). (c) The signal ∂S/∂n(n) at 3.2 K for Si-UW2 is shown with filled symbols: at zero field (black boxes),B||=5.5 T (blue triangles) and 9 T (red boxes). Empty symbols (right axis) are the corresponding effective masses atB=0 (black) andB||=9 T (red). The bars illustrate schematically the band diagram for two spin subbands in the regionsA,BandC. Vertical dashed lines depict schematic borders between the regionsA,BandC. (d) The entropy of the 2D electron system measured in Si-UW2 for three temperatures (symbols). Inset: temperature dependence of the entropy forn=10.5 × 1011cm−2(EF=75 K) and 3.9 × 1011cm−2(EF=30 K). Dashed curves denote the upper estimate for the entropy. Figure 2: Entropy per electron in zero perpendicular field. ( a ) The entropy per electron ∂ S /∂ n versus density (symbols) for various temperatures, sample Si-UW2. Inset: the same data versus dimensionless density ( E F / T ), the solid curve is the expectation for the Fermi gas with the Si band parameters, the dashed curve is the expectation for the FL with negative ∂ m */∂ n (see text); ( b ) the effective mass m * versus density. The black curve corresponds to the approximation of m * from the Shubnikov-de-Haas measurements [4] . Symbols are the m *( n , T ) data determined using equation (4) from the measured ∂ S /∂ n values. Different symbols correspond to different temperatures (shown in the inset). Scaling of the effective mass versus effective interaction parameter is shown in the inset(see text). ( c ) The signal ∂ S /∂ n ( n ) at 3.2 K for Si-UW2 is shown with filled symbols: at zero field (black boxes), B || =5.5 T (blue triangles) and 9 T (red boxes). Empty symbols (right axis) are the corresponding effective masses at B =0 (black) and B || =9 T (red). The bars illustrate schematically the band diagram for two spin subbands in the regions A , B and C . Vertical dashed lines depict schematic borders between the regions A , B and C . ( d ) The entropy of the 2D electron system measured in Si-UW2 for three temperatures (symbols). Inset: temperature dependence of the entropy for n =10.5 × 10 11 cm −2 ( E F =75 K) and 3.9 × 10 11 cm −2 ( E F =30 K). Dashed curves denote the upper estimate for the entropy. Full size image As we found, the mass m * extracted from our data in the FL regime agrees reasonably with the effective mass measured from damping of the amplitude of quantum oscillations [4] (for more detail, see Supplementary Note 6 ). As density decreases, the electron system inevitably enters the correlated plasma regime E F ≲ T < U for which the FL theory is inapplicable. There were experimental indications (see refs 17 , 18 , and Fig. 3 a,b of ref. 4 ) that electron–electron interactions preserve parabolic spectrum ɛ = p 2 /2 m * in the 2D Fermi-liquid in the wide energy range, rather than in the vicinity of the Fermi level. We expect therefore that even in the plasma regime, the entropy should carry signatures of the interaction-enhanced effective mass. Examples of the ∂ S /∂ n density dependence for several temperatures are shown in Fig. 2a . Qualitatively, the data is consistent with the above expectations: (i) the larger the temperature, the higher is the entropy (area under the curve); (ii) as the Fermi energy (electron density) increases, ∂ S /∂ n tends to zero and (iii) for the lowest temperatures and highest densities, ∂ S /∂ n becomes negative, in accord with that anticipated for the Fermi liquid. The inset of Fig. 2a shows that the experimental ∂ S /∂ n data are systematically higher than the theoretical dependence for noninteracting Fermi gas, calculated from equation (4) (with the bare band mass 0.19 m e ). Since the entropy is proportional to the density of states averaged over the energy interval T , we attribute such excessive entropy regions to the modified effective mass. Lacking a microscopic theory for non-degenerate strongly interacting electron system, we fitted our results using equation (4) with a density dependent effective mass m *( n ) as a fitting parameter. Thus extracted effective mass for different temperatures is shown in Fig. 2b . In the high temperature limit T ≳ U ≫ E F , the kinetic energy of electrons is given by temperature; hence, the 2D electron gas turns out to be weakly interacting and ∂ S /∂ n is expected to be described by equation (4) with the density-independent effective mass close to the band mass value m b . In general, for a given temperature, the effective mass exhibits a re-entrant behaviour: as density decreases m * first grows, then passes through a maximum and falls down approaching a value of the order of m b . The lower the temperature, the higher maximum value the effective mass reaches. The enhanced effective mass is in a qualitative agreement with the low-temperature Shubnikov-de-Haas measurements of ref. 4 (shown with a thick curve in Fig. 2b ). The low-density region, where the effective mass falls as density decreases, corresponds to a non-degenerate strongly correlated electron plasma regime ( E F ≲ T < U ). We are not aware of any theory describing this domain. To treat the data in this regime, we suggest the following phenomenological approach. For the degenerate clean 2D Fermi liquid, renormalization of its physical parameters, and, particularly, the effective mass, is governed by a single dimensionless variable equal to the ratio of the potential interaction energy U to the kinetic Fermi energy, (ref. 14 ). Here stands for the effective Bohr radius with average dielectric constant. As explained above, when temperature increases, the interactions for a given density weaken and cannot be characterized anymore by r s ∝ U/ E F . Correspondingly, to describe our m *( n , T ) data set over the wide range of densities and temperatures, we suggest a phenomenological effective interaction parameter which interpolates the two limits, of the degenerate Fermi liquid and non-degenerate correlated plasma. It appears that all nonmonotonic m *( n ) dependencies for various temperatures collapse onto a single curve, when we choose α =0.4, β =1 and γ =1 (see the inset in Fig. 2b ). Some supporting reasonings from the plasma physics can be found in Supplementary Note 7 , though the precision of our measurements is not too high to exclude other possible functional forms. Role of the in-plane magnetic field To have a deeper insight into the effective mass renormalization in the low-density regime, we repeat the same measurements with the in-plane magnetic fields B || =5.5, and 9 T, which produce Zeeman splitting E Z : 0.5 and 1 meV, respectively (see Fig. 2c ). At low densities ( E F ≲ T , region A in Fig. 2c ) the plasma is spin-polarized by B || =9 T. Therefore, both, S and ∂ S /∂ n at B || =9 T are expected to be less than the respective zero field values. Region A is located in the vicinity of the critical density for sample Si-UW2 ( n c ≈8 × 10 10 cm −2 ) and below it. If the free spins existed in the 2D system in the region A , as the Mott–Wigner scenario of the 2D MIT predicts [19] , they would be fully polarized by the magnetic field gμ B B > T (that is, at both B || =9 T and B || =5.5 T), and the entropy would fall significantly by n s ln2 (where n s is the density of the free spins). However, in 5.5 Tesla field ( gμ B B > T =3.2 K), there is only a small ( ∼ 10%) drop of the entropy per electron, which well corresponds to a partial polarization of itinerant electrons, as seen in Fig. 2c . To further show that the drop of entropy in parallel field is simply due to Zeeman polarization of the plasma, we extract the effective mass for the Fermi gas [using equation (4) for B =0 as it was done above and equation (8) from Supplementary Note 8 for the Zeeman field] from our B =0 and 9 Tesla ∂ S /∂ n data (see Fig. 2c ). The resulting mass is shown in Fig. 2c with empty symbols. In region A (plasma regime), the effective masses for B =0 and B =9 T agree with each other to within 10%, thus justifying our Fermi-plasma approach. In region C , for both B =0 and B =9 T cases, the system is almost Fermi-liquid, where as explained above ∂ S /∂ n should be negative and small. In the crossover (plasma to liquid) regime B, the ∂ S /∂ n signal changes sign ( Fig. 2c ). For 9 T field, the sign change happens at higher density than that for B =0; respectively, the extracted mass at 9 T exceeds essentially the one at zero field. Qualitatively, this is because the non-degenerate minority subband produces the gaseous-like large contribution to the 9 T data. The crossover regime requires more detailed consideration. In region C , the density of states and hence the entropy should be the same at 9 T and at zero field. This means that the total area under the ∂ S /∂ n curves in Fig. 2c should be the same. Indeed the hatched areas in Fig. 2c do compensate each other. Integration of entropy in zero field Integration of the ∂ S /∂ n signal from zero density produces the entropy shown in Fig. 2d . We neglect the low-density experimentally inaccessible domain n < n th because it may lead only to a slight shift of the result, as shown by the dashed lines in Fig. 2d . Plotting the extracted entropy as a function of temperature, we see that for high electron density ( n =1.03 × 10 12 cm −2 ) it develops linearly in T (see insert to Fig. 2d ), extrapolating to zero at zero temperature, as it should be for a FL according to the third law of thermodynamics. For lower density ( n =3.9 × 10 11 cm −2 ), the S ( T ) dependence does not extrapolate linearly to zero at T =0. It is possible that for this density, the low- T FL regime is not achieved yet, and for even lower temperatures S ( T ) should tend to zero with an increased slope, corresponding to the enhanced effective mass. Role of disorder To further elucidate whether the mass growth originates from interelectron interactions or from disorder, we performed similar measurements with a more disordered sample Si8-9 whose mobility is lower by a factor of six (see Fig. 3 and Supplementary Note 9 where transport data are shown). We note that sample Si8-9 shows no signatures of the metal-to-insulator transition. The threshold density in Si8-8 is much higher than in Si-UW2 (see inset in Fig. 3 ), therefore only the data above n =1.5 × 10 11 cm −2 are available. First, as well as for the high-mobility sample Si-UW2, the signal (∂ S /∂ n ) for Si8-9 exceeds considerably the expected signal for the Fermi gas (dashed lines in Fig. 3 ). Second, within the density range where data are available for both samples, they are close to each other for all the three temperatures. The above facts signify that the effective mass enhancement is disorder independent. 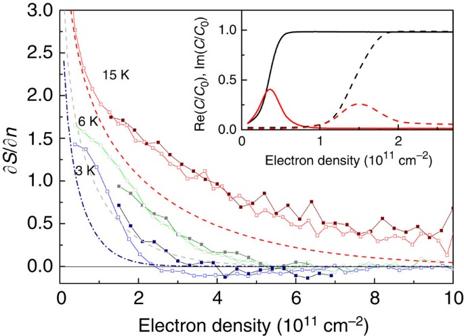Figure 3: Comparison of clean and disordered Si samples. Entropy per electron versus electron density in Si8-9 (filled symbols) and Si-UW2 (empty symbols) for three different temperatures (15 K—red colours, 6 K—grey colours, 3 K—blue colours). Theory expectation for ideal Fermi gas are shown by red dashed line(15 K), grey dotted line (6 K) and blue dash-dotted line(3 K). The inset shows real(black) and imaginary(red) components of capacitance taken at the ∂S/∂nmeasurement frequency for the clean sample Si-UW2 (solid lines) and disordered sample Si8-9 (dashed lines) respectively at 3 K. Figure 3: Comparison of clean and disordered Si samples. Entropy per electron versus electron density in Si8-9 (filled symbols) and Si-UW2 (empty symbols) for three different temperatures (15 K—red colours, 6 K—grey colours, 3 K—blue colours). Theory expectation for ideal Fermi gas are shown by red dashed line(15 K), grey dotted line (6 K) and blue dash-dotted line(3 K). The inset shows real(black) and imaginary(red) components of capacitance taken at the ∂ S /∂ n measurement frequency for the clean sample Si-UW2 (solid lines) and disordered sample Si8-9 (dashed lines) respectively at 3 K. Full size image Interestingly, the explored domain of low densities ( n <3 × 10 11 cm −2 ) and temperatures (2.5 K< T <5 K) belonging to the correlated plasma regime is exactly the regime of the strong ‘metallicity’ and the MIT for 2D electron systems in high-mobility Si-MOSFETs [2] , [5] . The observation that the domain of densities in the vicinity of the 2D MIT critical density falls into the strongly interacting plasma regime and can be parametrized with the temperature-dependent interaction parameter is novel for MIT physics. It points to the necessity of refining the existing theoretical approaches, because most of theoretical models [3] , [19] , [20] , [21] , [22] , [23] assume degenerate system. We note that our findings do not exclude quantum phase transition or divergency of the effective mass at even lower temperatures. It is worth noting here that everywhere we indirectly assume that our system is uniform down to the lowest densities. We can do so because we probe the 2D system on the (0.3–1)s timescale rather than the ps-scale as in transport measurements. For this reason, the regions (if any), poorly-conductive in transport, are well rechargeable in entropy measurements and the criteria of the inhomogeneity (that is a drop in the rechargeable area, that is, in the capacitance) is shifted deep to the lower density side. In our case for high-mobility Si samples, we do not observe drop of the capacitance down to half the critical density (see the insert to Fig. 3 ). This result is similar to that for n-GaAs in ref. 8 ) and therefore we believe that our system is relatively uniform, in the above sense and in the explored elevated temperature range. In Supplementary Note 10 , we give numerical arguments that the potential nonuniformity is not essential for thermodynamic ∂ S /∂ n measurements unless the sample fails to recharge. To summarize, to measure the equilibrium thermodynamic entropy of 2D electron systems, we developed the capacitive technique, whose sensitivity enables measurements with 10 8 electrons only. The key-feature of the method consists in measuring the entropy per electron, ∂ S /∂ n , rather than the heat capacitance c = T d S /d T as in the conventional AC calorimetry. We traced the entropy evolution in the wide ranges of electron density and temperature, from the low-temperature FL regime to the regime of non-degenerate strongly correlated electron plasma. We demonstrate that the plasma regime may be phenomenologically mapped to the ideal Fermi gas with a renormalized mass. To characterize the renormalization of the effective mass, we introduce an effective interaction parameter which is temperature and density dependent. Our experimental findings are challenging for the theory of the strongly correlated 2D plasma. Temperature modulation and measurements To modulate the temperature and to avoid its possible gradients, we used a copper cylindric sample holder of the diameter d =10–15 mm and the height h =4 mm with two r =100 Ohm twisted pair manganine heaters wound onto it. One heater was used to control the average temperature of the holder, the other was used for temperature modulation. The sample and thermometer were glued to the bottom of the holder with heat-conductive varnish. As a thermometer to detect the holder temperature, we used either Au:Fe–Cu thermocouple or RuO 2 chip resistor. The RuO 2 resistance was measured at elevated frequency ( ∼ 1,000 Hz) and then its modulation at the frequency f was detected with a separate lock-in amplifier. Entropy per electron measurements The signal ∂ S /∂ n was detected on a double heating current modulation frequency. For details concerning the choice of the frequency and explanation why the electrons are in thermal equilibrium with the sample, we refer to the Supplementary Note 1 . To measure femtoampere modulation current, a special care was taken to shield the sample from the heater, to ground the measurement circuit properly and to suppress vibrations. The scheme of the home-made amplifier (current-to-voltage converter) and the analysis of its operation are given in Supplementary Note 2 . Samples and characterization The parameters of the samples used are summarized in the Supplementary Table 1 . Electron density in the studied systems was determined by using either the low-field Hall effect or the magnetocapacitance dips in the quantum Hall Effect regime. Both methods give almost the same density value. See Supplementary Note 11 for details. For GaAs-gated heterojunctions, measurements and integration of ∂ S /∂ n in a wide range of densities were impossible because of extremely large equilibration times and pA-level leakage in Schottky-gate at low densities (high negative gate voltages). Theoretical background All required theoretical basis is summarized in Supplementary Note 8 (2D systems in zero magnetic field) and Supplementary Note 4 (2D systems in finite magnetic field). How to cite this article : Kuntsevich, A. Y. et al. Strongly correlated two-dimensional plasma explored from entropy measurements. Nat. Commun. 6:7298 doi: 10.1038/ncomms8298 (2015).